Numerical processing in the human parietal cortex during experimental and natural conditions Human cognition is traditionally studied in experimental conditions wherein confounding complexities of the natural environment are intentionally eliminated. Thus, it remains unknown how a brain region involved in a particular experimental condition is engaged in natural conditions. Here we use electrocorticography to address this uncertainty in three participants implanted with intracranial electrodes and identify activations of neuronal populations within the intraparietal sulcus region during an experimental arithmetic condition. In a subsequent analysis, we report that the same intraparietal sulcus neural populations are activated when participants, engaged in social conversations, refer to objects with numerical content. Our prototype approach provides a means for both exploring human brain dynamics as they unfold in complex social settings and reconstructing natural experiences from recorded brain signals. The foundation of our scientific practice rests upon the measurements we make during experimental paradigms in which the influence of the natural environment is reduced as much as possible, with all variables and confounds being eliminated or kept to a bare minimum. By contrast, real life is always shaped by ever-changing environmental factors and flowing social interactions, which have made it near impossible to study brain dynamics as they unfold in natural conditions. Recent neuroimaging studies have broken new ground for deciphering hemodynamic brain responses during relatively more naturalistic conditions such as watching a movie, listening to a story or viewing a visual scene inside the scanner [1] , [2] , [3] , [4] , [5] , [6] , [7] , [8] , [9] , [10] . Yet, despite these advances, functional imaging studies have inherent limitation in decoding brain activity within the subject’s own environment. These methodological factors have limited imaging-based investigations to behaviourally passive states during the experimental presentation of natural stimuli within the scanner. Electrophysiological studies with scalp electroencephalography (EEG), on the other hand, have been shown to be suitable for recordings in natural conditions [11] , [12] , [13] , [14] , [15] , [16] , [17] . However, given the limitation of scalp EEG in localizing the precise source of electrical signals, we relied on intracranial recordings to capture brain responses from populations of neurons during experimental as well as natural conditions. We designed the current study to measure focal brain activity during a well-established experimental condition before examining the activity of the same brain region during natural conditions. For this, we focused on numerical processing, which represents one of the more complex cognitive functions of the association areas of the human brain. Extant neuroimaging evidence in humans and electrophysiological studies in non-human primates have shown increased activation within the intraparietal sulcus (IPS) region during experimental conditions of numerosity [18] , [19] , [20] , [21] . However, intracranial electrophysiological studies of the IPS in humans during similar conditions have been missing. It has also been entirely unknown if a given IPS neuronal population responds to events with numerical content during natural conditions. We used electrocorticography (ECoG) in patients with epilepsy, who were implanted with chronic intracranial electrodes covering the lateral parietal lobe for ~7–10 days, during which simultaneous video monitoring was performed. In combination, this unique set of simultaneous ECoG/video data allows for anatomically precise recordings from the human brain during free behaviour. Each recording ECoG electrode captures electrophysiological signals from a population of neurons (~500,000 cells) with high anatomical precision and temporal resolution [22] . These electrodes are implanted chronically for several days and the activity in a precise location of the brain can be studied during spontaneous social interactions. Although the ECoG electrodes capture oscillatory signals in several narrow band rhythms such as α -, θ- or γ -bands, our focus was on changes of high-frequency broadband (HFB) activity also known as high- γ . Unlike synchronous oscillatory rhythms, HFB activity reflects asynchronous summation of population firing [22] and directly correlates with blood-oxygenation-level-dependent (BOLD) activity [23] , [24] , [25] . Given the evidence from prior studies showing strong BOLD responses in the human IPS during numerical cognition tasks and those suggesting a direct link between HFB activity and increased BOLD response, we focused our current analysis to test the following two hypotheses. First, that there is higher HFB response in the IPS during experimental arithmetic condition compared with non-arithmetic conditions; and second, that the same IPS area will show increased HFB response during periods of numerical processing in natural conditions. To test the two hypotheses, we conducted a controlled experiment in three patients with intracranial recordings. Participants performed a controlled experiment twice in which they were instructed to judge the accuracy of complete arithmetic equations and non-arithmetic memory statements ( Fig. 1a ). We established, in each individual participant’s brain, the parietal areas with significant HFB activity during the experimental arithmetic condition. Next, we selected these same anatomical locations and retrospectively explored simultaneous ECoG and video recordings to study the behavioural correlates of HFB activity during natural conditions, that is, when patients were engaged in everyday activities. We report here that a set of neuronal populations within the human IPS show increased HFB activity during the experimental arithmetic condition, and that the same neuronal populations are activated when participants, engaged in social conversations, refer to objects with numerical content. Our approach provides a means for both the exploration of human brain dynamics as they unfold in complex social settings and the reconstruction of naturalistic experiences from brain signals. 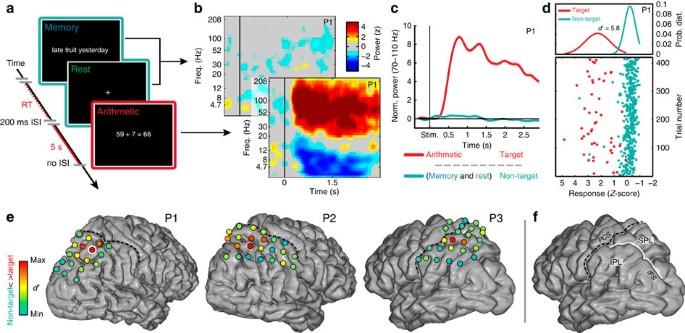Figure 1: ECoG responses in the human IPS region during experimental arithmetic condition. The experimental task (a) consisted of self-paced arithmetic (simple addition equations) and non-arithmetic conditions (memory statements and 5-s fixation). During the arithmetic condition, we found a significant increase of activity in some but not all electrodes. As seen in the time-frequency plot (b), this activity was best measured in the high-frequency broadband (HFB, 70–110 Hz) range. The temporal profile of relative HFB power changes (c) are shown for one representative electrode (P1–1) averaged across trials. Usingd′-values, the separation of the distributions of HFB responses during arithmetic (red, target) and non-arithmetic (blue, non-target) conditions (d) could be quantified. In each participant’s brain, thed′-values were mapped (e), and the sites with the highestd′-values (red) were located around the IPS region (white line inf). The IPS divides the superior (SPL) from the inferior parietal (IPL) lobules. PCS (post central sulcus) is shown with dashed line. Among all subjects, electrode P1–1 (red electrode with white circle ine) had the highestd′-value. Figure 1: ECoG responses in the human IPS region during experimental arithmetic condition. The experimental task ( a ) consisted of self-paced arithmetic (simple addition equations) and non-arithmetic conditions (memory statements and 5-s fixation). During the arithmetic condition, we found a significant increase of activity in some but not all electrodes. As seen in the time-frequency plot ( b ), this activity was best measured in the high-frequency broadband (HFB, 70–110 Hz) range. The temporal profile of relative HFB power changes ( c ) are shown for one representative electrode (P1–1) averaged across trials. Using d′ -values, the separation of the distributions of HFB responses during arithmetic (red, target) and non-arithmetic (blue, non-target) conditions ( d ) could be quantified. In each participant’s brain, the d ′-values were mapped ( e ), and the sites with the highest d ′-values (red) were located around the IPS region (white line in f ). The IPS divides the superior (SPL) from the inferior parietal (IPL) lobules. PCS (post central sulcus) is shown with dashed line. Among all subjects, electrode P1–1 (red electrode with white circle in e ) had the highest d ′-value. Full size image Demographics and brain coverage Formal clinical neuropsychological evaluations suggested that the three participating patients were all right-handed individuals with normal IQ. The three participants were P1 (female), P2 (male) and P3 (male). Across the three participants, grids of electrodes covered the left (112 electrodes) or the right (178 electrodes) hemispheres. The location of the grids was determined by clinical needs, and the seizure foci were found to be in the right medial parietal (P1), right medial occipital (P2) and left insular (P3) cortices. The lateral parietal coverage was necessary for clinical purposes, but only after intracranial monitoring it was found to be void of epileptic activity. Using the anatomical boundaries as defined in Fig. 1 , we found 65 parietal electrodes (P1=18, right; P2=23, right; P3=24, left) that covered the anatomical landmarks of the lateral parietal cortex (LPC) and were free of any epileptic or artefact activity. Behavioural data Each participant performed the experimental task twice and the behavioural data were largely consistent across sessions ( Table 1 ). Participants performed significantly above chance level in both sessions, except for participant P3 who performed relatively poorly during the first but improved his performance during the second session of the same experiment. The arithmetic trials constituted ~20% of the task duration ( Table 1 ). Table 1 Behavioural data. Full size table HFB power in IPS discriminates the numerical condition We evaluated the response of each parietal electrode in all frequency bands by their event-related spectral perturbation (ERSP) for all conditions and measured their temporal response profiles in six distinct bands of activity: δ (1–4 Hz), θ (4–8 Hz), α (8–12 Hz), β (15–25), low- γ (30–55 Hz), and a relatively narrower band of HFB (70–110 Hz) was chosen to avoid line noise. This analysis revealed a lack of significant increase of power, during the arithmetic condition, in the lower bands across the 65 parietal electrodes (P1=18, P2=23 and P3=24). However, in 20 electrodes (P1=10, P2=8 and P3=2), we found a significant increase of power in the HFB range during this condition (Student’s t -test, P <1.6 × 10 −4 , Bonferroni corrected). In light of this significant difference, we then estimated the degree of separation between conditions. We found that 14 of these HFB-activated electrodes (P1=7, P2=5 and P3=2) had d ′-values greater than 0.75 (unit of s.d.). In other words, 20 electrodes had statistically distinct distributions for arithmetic and non-arithmetic conditions (using P -values), but in only 14 of these electrodes the two distributions were distinct from each other (using d ′-values). Interestingly, the electrodes with the most significant increase of HFB activity during the arithmetic condition and with the highest d ′-values were all located within the IPS ( Fig. 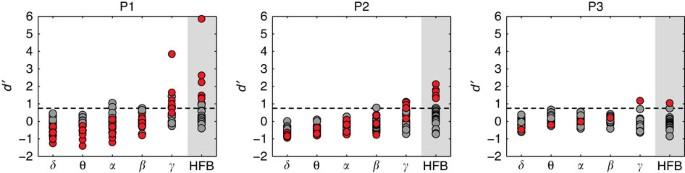Figure 2: Thed′-values of response in different frequency bands during the arithmetic condition. The three plots show thed′-values (vertical axis) of parietal electrodes in different frequency ranges (horizontal axis) in participants P1, P2 and P3. The horizontal dashed line represents thed′-value of 0.75 (the higher thed′-values, the more selective activity during the experimental arithmetic condition). Each dot represents one electrode selected to be within the anatomical boundaries of the parietal lobe. Electrodes with significant increase of HFB activity during the experimental arithmetic condition are filled in red. Interestingly, none of these electrodes showed increase of activity in lower frequency bands during the arithmetic condition. 1f —for MNI coordinates of these electrodes see Table 2 ). Table 2 The d ′-values for the HFB peaks and the MNI coordinates of the electrodes. Full size table Importantly, the power of response in δ- , θ -, α - or β -bands was not increased significantly in any of the 14 electrodes and their d ′-values were low ( d ′<0.34, P >0.03, Bonferroni corrected for number of electrodes and conditions, df=416 (n1=48 and n2=370), two-sample, right-tailed Student’s t -test, Fig. 2 ). The power of low- γ band was significantly increased in P1 ( n =3 electrodes, d ′>1.2, P <10 −14 ) and P3 ( n =1, d ′=1.18, P =2.7 × 10 −13 ) and the d ′-values were high. Figure 2: The d ′-values of response in different frequency bands during the arithmetic condition. The three plots show the d ′-values (vertical axis) of parietal electrodes in different frequency ranges (horizontal axis) in participants P1, P2 and P3. The horizontal dashed line represents the d ′-value of 0.75 (the higher the d ′-values, the more selective activity during the experimental arithmetic condition). Each dot represents one electrode selected to be within the anatomical boundaries of the parietal lobe. Electrodes with significant increase of HFB activity during the experimental arithmetic condition are filled in red. Interestingly, none of these electrodes showed increase of activity in lower frequency bands during the arithmetic condition. Full size image As noted, the same experimental task was administered twice in each participant with identical but randomly ordered trials. We used the first session as the ‘training session’ to establish optimal with HFB amplitude and duration parameters for detection of arithmetic trials in the second session, that is, the ‘testing session’. For this, we relied on receiver-operating characteristic curves (ROCs, Fig. 3a–c ). These optimal parameters identified the supra-threshold events that we labelled as ‘HFB peaks’. We evaluated the sensitivity and specificity of the HFB peaks in separating arithmetic (target) from non-arithmetic (non-target) trials in the testing session and found that both sensitivity and specificity of the HFB peaks in training sessions were similar to the ones obtained during the testing session ( Fig. 4 ). Given that the training and testing sessions were recorded at different times, the stability of the results from training to testing session suggested that the statistics of the signals were qualitatively stable (that is, positively skewed and leptokurtotic) and did not change significantly over time. Using HFB peaks as events of interest enabled us to make discrete signals from the instantaneous amplitude fluctuation and subsequently in each electrode determine a ‘selectivity index’ for the arithmetic condition during the testing session. We found that all of the 14 arithmetically responsive electrodes had a high selectivity index (>0.25) and, more importantly, electrodes with higher d ′-values also had higher selectivity ( r =0.8, P =0.007, Pearson’s correlation, Fig. 5a ). It should be noted that the selectivity index values were extracted from the experimental trial-by-trial analysis whereas the d ′-values were calculated from the continuous analogue HFB trace. Therefore, this analysis established a meaningful connection between the discrete signal in the experimental condition and the continuous analogue signal in the natural condition. It also confirmed that the measure of ‘HFB peak’ in the natural condition preserves the selective property of the HFB signal. 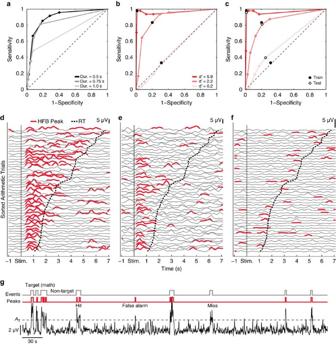Figure 3: Establishing optimal parameters for detecting HFB peak events. ROC curve inais from electrode P1–2 and the three lines are for three different duration parameters (0.5, 0.75 and 1.0 s). Each dot on the lines represents a given amplitude threshold. For the optimal duration parameter 0.5 s (black line), the best amplitude threshold is the one with maximal specificity and sensitivity values, that is, closest to the top left. The ROC curve inbis for three adjacent electrodes in P1 with three differentd′-values. Electrode P1–1 (marked inFig. 1e) had the highestd′-value of 5.9. The electrode immediately anterior to this, had a lesserd′-value of 2.2 (same ROCs as ina). The electrode immediately posterior to P1–1 had ad′-value of 0.2. The position of these electrodes are shown inFig. 1e, P1. The ROC curve of the electrode P1–1 is closest to the top left corner with highest sensitivity and specificity values. In contrast, the ROC curves of the electrode with minimumd′-value lies almost on the diagonal line. The ROC incshows the values from training and testing sessions in the same three adjacent electrodes as inb. Parameters from the training and testing sessions gave very similar results (hollow and filled markings). Data ind–fare for the same three electrodes as inbandc, showing the sorted arithmetic trials in electrodes withd′-values of 5.9 (d), 2.2 (e) and 0.2 (f). All arithmetic trials were sorted based on their durations and aligned with respect to the stimulus onset (black vertical line.) The participant’s button-press was marked by the dashed curved line followed by the next trial. Continuous HFB power fluctuation along with the HFB peaks and continuous sequence of arithmetic and non-arithmetic trials in a 5-min recording are shown ing. The HFB peaks (red) marked the significant increase in the HFB power that co-occurred during arithmetic trials (hit) and non-arithmetic trials (false alarm). Figure 3: Establishing optimal parameters for detecting HFB peak events. ROC curve in a is from electrode P1–2 and the three lines are for three different duration parameters (0.5, 0.75 and 1.0 s). Each dot on the lines represents a given amplitude threshold. For the optimal duration parameter 0.5 s (black line), the best amplitude threshold is the one with maximal specificity and sensitivity values, that is, closest to the top left. The ROC curve in b is for three adjacent electrodes in P1 with three different d ′-values. Electrode P1–1 (marked in Fig. 1e ) had the highest d ′-value of 5.9. The electrode immediately anterior to this, had a lesser d ′-value of 2.2 (same ROCs as in a ). The electrode immediately posterior to P1–1 had a d ′-value of 0.2. The position of these electrodes are shown in Fig. 1e , P1. The ROC curve of the electrode P1–1 is closest to the top left corner with highest sensitivity and specificity values. In contrast, the ROC curves of the electrode with minimum d ′-value lies almost on the diagonal line. The ROC in c shows the values from training and testing sessions in the same three adjacent electrodes as in b . Parameters from the training and testing sessions gave very similar results (hollow and filled markings). Data in d – f are for the same three electrodes as in b and c , showing the sorted arithmetic trials in electrodes with d ′-values of 5.9 ( d ), 2.2 ( e ) and 0.2 ( f ). All arithmetic trials were sorted based on their durations and aligned with respect to the stimulus onset (black vertical line.) The participant’s button-press was marked by the dashed curved line followed by the next trial. Continuous HFB power fluctuation along with the HFB peaks and continuous sequence of arithmetic and non-arithmetic trials in a 5-min recording are shown in g . The HFB peaks (red) marked the significant increase in the HFB power that co-occurred during arithmetic trials (hit) and non-arithmetic trials (false alarm). 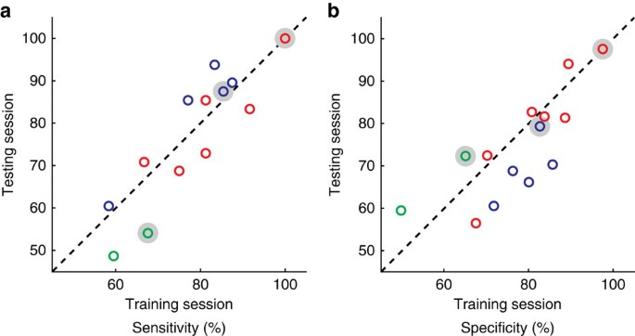Figure 4: Sensitivity and specificity values in training and testing sessions. Parameters from the training session produced similar results on the testing session; the sensitivity (a) and specificity (b) values obtained from applying parameters from the first session (training session) and from the second session (testing session) were similar (close to diagonal line where two values are identical). Each point indicates an electrode from participants P1 (red), P2 (blue) and P3 (green). Full size image Figure 4: Sensitivity and specificity values in training and testing sessions. Parameters from the training session produced similar results on the testing session; the sensitivity ( a ) and specificity ( b ) values obtained from applying parameters from the first session (training session) and from the second session (testing session) were similar (close to diagonal line where two values are identical). Each point indicates an electrode from participants P1 (red), P2 (blue) and P3 (green). 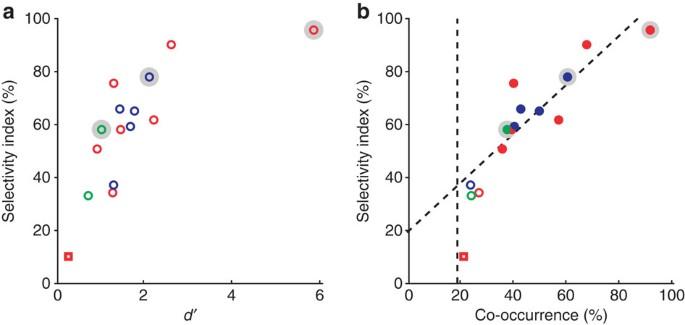Figure 5: Selectivity and co-occurrence of HFB activity. In both panels, markers in red, blue and green represent electrodes from participants P1, P2 and P3, respectively. For each participant, the electrode with the highestd′-value is marked with a shaded halo. The red square marker in each plot represents the control electrode also shown inFig 2f. (a) Selectivity index values increase in parallel withd′-values (n=14, Spearman’s rank correlation,r=0.8,P=0.0007). (b) Co-occurrence values for the HFB increase in the experimental condition are also correlated with the selectivity index values. Electrodes with higher selectivity index during experimental condition showed higher co-occurrence of HFB peaks during experimental arithmetic condition (n=14, Pearson’s correlation,r=0.9,P=1e−5). Full size image Figure 5: Selectivity and co-occurrence of HFB activity. In both panels, markers in red, blue and green represent electrodes from participants P1, P2 and P3, respectively. For each participant, the electrode with the highest d ′-value is marked with a shaded halo. The red square marker in each plot represents the control electrode also shown in Fig 2f . ( a ) Selectivity index values increase in parallel with d ′-values ( n =14, Spearman’s rank correlation, r =0.8, P =0.0007). ( b ) Co-occurrence values for the HFB increase in the experimental condition are also correlated with the selectivity index values. Electrodes with higher selectivity index during experimental condition showed higher co-occurrence of HFB peaks during experimental arithmetic condition ( n =14, Pearson’s correlation, r =0.9, P =1e−5). Full size image Furthermore, we defined the so-called ‘co-occurrence’ value as the ratio of the number of HFB peaks during the arithmetic condition to the total number of HFB peaks. We found that the co-occurrence values were significantly beyond the chance level for electrodes ( n =14) with high selectivity index ( r =0.9, P =0.00001, Pearson’s correlation, Fig. 5b ). HFB activity in IPS during natural conditions Once we determined the optimal parameters, we applied the same parameters and identified the HFB peaks in the ECoG data during the natural condition ( Fig. 6 ). First, we determined the exact times at which these HFB peaks occurred during the natural condition. In parallel, and in a blind manner, independent raters watched the video files recorded simultaneously with the ECoG data, and determined the exact times at which behavioural events of interest occurred. These included conversations of words or viewing of objects with numerical content in space, time or magnitude. We then analysed the timing of these behavioural events with the timing of the HFB activity ( Fig. 7 and Supplementary Movie 1 ). This analysis revealed two important findings. 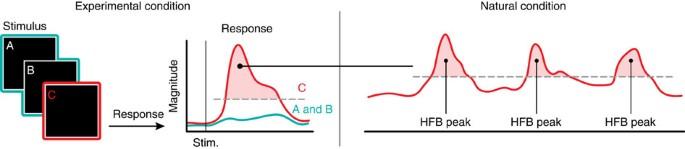Figure 6: From experimental to natural conditions. In the controlled experimental task (a), neural responses during the target condition of interest (condition C, red) was compared with control conditions (conditions A and B, green). We defined optimal discriminating duration and amplitude parameters to separate the target condition C from the mixture of conditions A and B in the experimental data. We applied the same optimal parameters to the spontaneous ECoG data acquired during the natural condition (b) and detected discrete events (that is, HFB peaks) during which the HFB power was increased. Figure 6: From experimental to natural conditions. In the controlled experimental task ( a ), neural responses during the target condition of interest (condition C, red) was compared with control conditions (conditions A and B, green). We defined optimal discriminating duration and amplitude parameters to separate the target condition C from the mixture of conditions A and B in the experimental data. We applied the same optimal parameters to the spontaneous ECoG data acquired during the natural condition ( b ) and detected discrete events (that is, HFB peaks) during which the HFB power was increased. 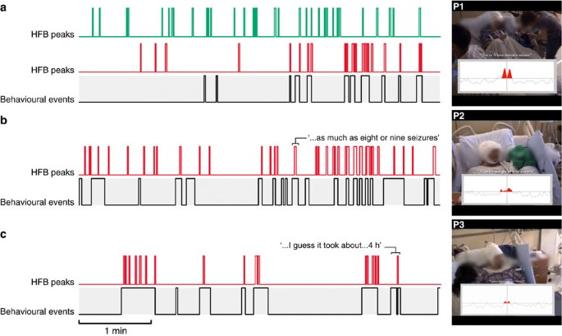Figure 7: HFP peaks in the natural condition. Traces show the occurrence of HFB peaks and behavioural events of interest in the natural condition in the three participants P1 (a), P2 (b) and P3 (c). The green trace inais from a control parietal electrode (the same as inFig. 2e), whereas the red traces are from the electrode with the highestd′-values in each participant. There is a remarkable co-occurrence between behavioural events and HFB peaks in red traces but not the green trace. The behavioural events overwhelmingly involve expressions counting objects, individuals, quantities, amounts, times and events in an ordered sequence. This includes all numerals, ordinals and quantifiers (for example, ‘some’, ‘all’ and ‘every’) when these combine with numerals or quantities, as well as some other expressions (‘bunch of people’, ‘a bottle of coke’ and ‘extra little bit’). SeeSupplementary Movie 1. Full size image Figure 7: HFP peaks in the natural condition. Traces show the occurrence of HFB peaks and behavioural events of interest in the natural condition in the three participants P1 ( a ), P2 ( b ) and P3 ( c ). The green trace in a is from a control parietal electrode (the same as in Fig. 2e ), whereas the red traces are from the electrode with the highest d ′-values in each participant. There is a remarkable co-occurrence between behavioural events and HFB peaks in red traces but not the green trace. The behavioural events overwhelmingly involve expressions counting objects, individuals, quantities, amounts, times and events in an ordered sequence. This includes all numerals, ordinals and quantifiers (for example, ‘some’, ‘all’ and ‘every’) when these combine with numerals or quantities, as well as some other expressions (‘bunch of people’, ‘a bottle of coke’ and ‘extra little bit’). See Supplementary Movie 1 . Full size image First, electrodes that had shown significant increase of HFB activity during the experimental arithmetic condition exhibited only infrequent HFB peaks in the natural condition, even though the participants were involved in behaviours requiring attention, memory, language and purposeful eye and hand movements. In other words, the IPS neuronal populations identified to be involved in numerical cognition were not activated when participants moved their eyes or hands and grasped objects or paid attention to different parts of the space. To quantify this, we relied on the measure of ‘sparseness value’. In the controlled experimental design, one has a priori knowledge about which trials are arithmetic and which ones are non-arithmetic, and the ratio of hits over misses (and, therefore, selectivity index values) can be easily calculated. However, the natural condition does not have the trial-based structure of an experimental condition. Therefore, it is not amenable for the analysis of selectivity index. Instead, considering each HFB peak as a discrete event allowed us to calculate the sparseness value of response during the natural condition. This analysis, which related a property from the controlled experimental condition to another in the natural condition, showed that the sparseness values of HFB peaks correlated strongly with the selectivity index values of HFB during the experimental condition ( n =14, r =0.7, P =0.003, Fig. 8a ). Interestingly, the sparseness values of the HFB peaks varied across sites in the LPC and were highest in the IPS recording sites. 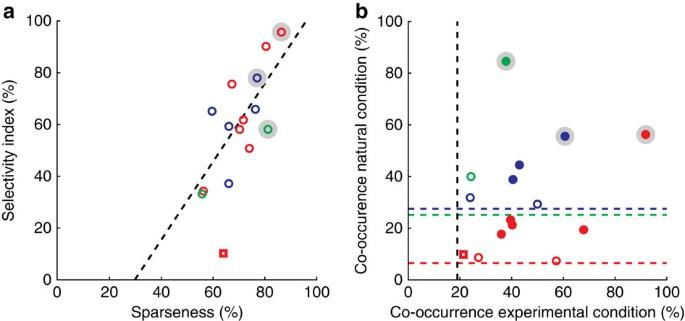Figure 8: Sparseness and selectivity index are related to co-occurrence values. In both panels, markers in red, blue and green represent electrodes from participants P1, P2 and P3, respectively. For each participant, the electrode with the highestd′-value is marked with a shaded halo. The red square marker in each plot represents the control electrode also shown inFig 2f. (a) Activity of electrodes responsive during experimental numerical condition was sparse during natural condition. The selectivity index and sparseness were correlated (Pearson’s correlation,n=14,r=0.7,P=0.0025). (b) Co-occurrence of HFB peaks during experimental numerical condition and natural numerical processing are correlated. HFB peaks co-occurred with numerical events greater than the chance level (shown with dashed lines) and this was significant for 9 out of 14 electrodes (filled markers,P<0.05). Figure 8: Sparseness and selectivity index are related to co-occurrence values. In both panels, markers in red, blue and green represent electrodes from participants P1, P2 and P3, respectively. For each participant, the electrode with the highest d ′-value is marked with a shaded halo. The red square marker in each plot represents the control electrode also shown in Fig 2f . ( a ) Activity of electrodes responsive during experimental numerical condition was sparse during natural condition. The selectivity index and sparseness were correlated (Pearson’s correlation, n =14, r =0.7, P =0.0025). ( b ) Co-occurrence of HFB peaks during experimental numerical condition and natural numerical processing are correlated. HFB peaks co-occurred with numerical events greater than the chance level (shown with dashed lines) and this was significant for 9 out of 14 electrodes (filled markers, P <0.05). Full size image Second, the infrequent HFB peaks in the natural condition occurred at the times when the participant read, heard or spoke words with numerical content (quantified by the co-occurrence value, Fig. 8b ). For each participant, neuronal populations with the highest d ′-values and the highest selectivity index during the experimental arithmetic condition had the highest co-occurrence values during both experimental and natural conditions, and were located around the IPS region (marked with shaded circles in Fig. 8 ). However, it should be noted that some neuronal populations with higher co-occurrence values during the controlled experimental condition did not have equally high co-occurrence values during the natural condition. This indicates that not all neuronal populations that were activated during explicit calculation showed an equally high degree of response during, for instance, the mere mention of numerical words. Moreover, the co-occurrence values changed significantly across neighbouring electrodes, suggesting that the functional correlate of the response was anatomically specific. For instance, three electrodes within a 2-cm range of the LPC in P1 had widely different co-occurrence rates ( Supplementary Table S1 , and Fig. 7a , green trace versus red trace). These quantitative findings aside, Supplementary Movie 1 clearly depicts the essence of IPS activation during naturalistic conditions. As seen in this video, neuronal populations with selective response to arithmetic stimuli during the experimental task exhibited HFB activity across different domains of numerical calculation and enumeration. For example, supra-threshold increases in HFB activity were seen during events ranging from the visual identification of numbers (Ishihara test) to enumeration of objects or individuals (for example, ‘a bottle of coke’, ‘some more Vicodin’, ‘another small group’, ‘bunch of people’, ‘extra little bit’, ‘some of the nurses’ and ‘all the nurses’, as well as estimation in the temporal domain (for example, ‘once every hour’, ‘the first night’, ‘every hour on the hour’, ‘10 days ago’ and ‘the day after last Monday’). The HFB peaks occurred during expressions of counting objects, individuals, quantities, amounts, times and events. This included numerals, ordinals and quantifiers (for example, ‘some’, ‘all’ and ‘every’) when they were combined with quantities or numbers (for example, ‘some sleep’, ‘all the nurses’ and ‘every two or three hours’), but not otherwise (for example, ‘some kind of research’, ‘all the time’ or ‘everything’). Real-life experience has a rich and constantly changing context that is shaped by the natural environment and human interactions, making it challenging to study the underlying brain activity during natural conditions. In this study, we have for the first time addressed the link between the activity of a specific neuronal population in the human brain during a controlled experimental condition and the activity of the same population of neurons during natural conditions. Our methodological advantage is directly related to the power of intracranial recording with ECoG in three domains: (1) anatomical precision of the recorded data, (2) temporal resolution of the signals and (3) the suitability of the method for chronic recordings during natural conditions. Our findings highlight the relevance and practical value of intracranial HFB signal as the best metric of localized cortical activation because of its striking spatial as well as functional selectivity [26] , [27] , [28] , [29] , [30] , [31] , [32] , [33] , [34] , [35] , [36] . We are mindful that the profile of recorded electrophysiological activity is rich and contains slower bands of activities (for example, α - or θ -band), but we found that the changes in the slow rhythmic bands of activity were not regionally or conditionally selective. Of additional note, low frequency changes in power show greater frequency variability across the brain, that is, some regions dominate in θ -power, whereas others have α - and β -canonical oscillations [29] , [37] . In contrast, the HFB signal provides a region-invariant measure of local neuronal activation. For instance, we show in the current study that the HFB power in the IPS is significantly increased during arithmetic processing and unchanged during episodic memory retrieval. In contrast, we recently showed a reverse pattern of HFB response in another region of the brain, that is, the posteromedial cortex, when subjects participated in the same experimental task that was used in the current study [29] , [38] . The posteromedial cortex showed an increase in the HFB response during memory retrieval but a sustained suppression of HFB response during arithmetic calculation. In other words, a given cognitive condition may cause different HFB responses in different cortical areas, depending on their level of engagement or disengagement in the cognitive condition. In our study, we used peaks of HFB power, that is, the ‘HFB peaks’ as a signature of discrete events that could be detected in continuous natural recordings. By using the same parameters for the HFB peaks that we had defined in the experimental condition, we were able to detect significant discrete events of instantaneous amplitude fluctuations during a continuous recording and explore the behavioural correlates for such discrete events retrospectively. By introducing this new approach, and because of the advantages of the ECoG method, we were able to compare the neuronal population activity in the human IPS during a controlled experimental arithmetic condition with the activity of the same neuronal population during natural conditions. The natural events that triggered the occurrence of HFB peaks involved seeing, hearing or expressing numerals, ordinals and quantifiers when these were combined with quantities or numbers. In line with clinical observations [39] , [40] , previous experimental neuroimaging studies have shown the involvement of the LPC in processing quantifiers [41] . For instance, comprehension of numerical quantifiers that require magnitude processing (for example, ‘at least three’) depends on a lateral parietal network, whereas the comprehension of logical quantifiers that require a simple form of perceptual logic (for example, ‘some’) does not [42] . Our findings suggested that the HFB responses in the IPS occurred after hearing words with numerical content or seeing numbers, and before the expression of words with numerical content. Most of the HFB peaks appeared early during speech production. The temporal lag or lead of HFB responses relative to behavioural events could not be precisely analysed for several reasons: First, in natural conditions, it is difficult to determine when exactly a participant thinks of a numerical concept before expressing it. Second, the duration of HFB peaks in our study was set to be at least 500 ms and this sets a lower bound on our temporal precision. Third, correlating the HFB peak timing with the time of behavioural response, one is limited by the sync offset between electrophysiological and video data. In our recordings, the maximum sync offset was ~200 ms. These limitations can be partially overcome in future studies with prospective design. Our study provides the first intracranial electrophysiological data in humans supporting the important role of the IPS region in numerical cognition. Moreover, our observations suggested a surprisingly high degree of sparseness of activity in the numerically responsive IPS neuronal populations during the natural condition. Although these populations of neurons showed a high degree of selectivity for the experimental condition of numerosity, they exhibited a great sparseness of HFB response during the natural condition when the participants were engaged in activities such as attending to visual objects in the room, recalling past memories, grasping and reaching movements, or saccades — activities that are known to activate the LPC. The selective and sparse activity in the IPS neuronal populations provides direct evidence that these populations have a specific role in numerical cognition rather than being co-opted during various other parietal functions. Future prospective studies are needed to confirm this assertion by measuring neuronal responses pertaining to various parietal functions during experimental as well as natural conditions. It should be noted that the aim of our retrospective study was not to catalogue various natural correlates of activity in various sites of the human parietal cortex. Similarly, our study was not designed to decipher the nature of numerical processing in the IPS region. For this, prospective well-designed studies with a denser array of electrodes are needed to differentiate distinct roles of adjacent neuronal populations in different aspects of numerical processing. Our observations provide interesting preliminary findings for such prospective studies. For instance, future studies are needed to decipher how specific IPS neuronal populations are engaged during explicit calculation versus implicit processing of numerical information. In these future studies, it will be important to determine whether the same IPS neuronal populations are involved in both explicit and implicit numerical processing and whether their activity is related to procedural problem solving. In our current study, we found that of 14 parietal electrodes the ones with the highest co-occurrence values during the controlled experiment also had the highest co-occurrence values during the natural condition. In other words, if an electrode’s HFB activity occurred more during calculation than in experimental memory and rest conditions, its HFB response in the natural condition was seen more during utterance of words with numerosity content than any other condition. More importantly, however, not every one of the 14 electrodes had the same co-occurrence match between experimental and natural conditions. Some with activity during experimental calculation condition showed significantly less response during the natural events with implicit numerosity processing and vice versa. It is possible that this mismatch between experimental and natural conditions reflects a difference in neuronal response to explicit versus implicit numerosity processing, depending on the anatomical location of the electrodes. In future studies, it will also be important to know how the activity of these IPS neuronal populations is related to the activity of other parietal and prefrontal areas, and rooted in procedural problem solving, and how it is subject to evolutionary and developmental changes [19] , [43] , [44] , [45] , [46] , [47] , [48] , [49] . In the same line, it will be important to explore the temporal and causal links between the activity of neuronal populations in the IPS and the ones in the inferior parietal lobule and the medial temporal lobes that are important for retrieval of mathematical knowledge [20] . We believe that our study also serves as a prototype for developing more sophisticated methods in the future. As others have demonstrated, online tools to detect localized brain responses [50] , [51] , [52] , [53] will have clinical use in functional mapping of the brain as well as in brain–machine interface paradigms, that is, cognitive neural prosthetics [54] , [55] . In theory, it may be possible to use our method to identify neuronal populations that are responsive during a given specific thought and be able to read the mind of a human individual. In parallel to such methodological advancements, new ethical issues may have to be addressed by neuroscience and law communities [56] , [57] , [58] . Participants Three patients were implanted with intracranial electrodes covering the lateral parietal surface on the right (participant 1, 64 electrodes and participant 3, 114 electrodes) or left (participant 2, 112 electrodes; Fig. 1 ). All three patients were implanted solely for clinical reasons and gave their informed consent to participate in the study, which was approved by the Stanford University Institutional Review Board. All patients were right handed, with normal IQ, with age 37, 43 and 45 years. In all participants, the lateral parietal electrodes of interest were void of pathological activity. Participant 1 was female and participants 2 and 3 were male. We emphasize that the aim of the current study was not to explore the lateralization of response or the effect of gender in numerical cognition, and thus our participants were not balanced on the basis of hemisphere coverage or gender. Experimental task and stimuli In the experimental task, participants judged with self-paced responses the accuracy of addition equations or memory statements. In the ‘arithmetic condition’, simple addition equations comprises adding one single digit with one double-digit number ( n =48). These equations were randomly mixed with the ‘non-arithmetic condition’, which contained the memory statements without any numerical content ( n =~258) and 5-s long fixation or rest trials ( n =~32). The task was administered twice in each participant (either the same day (P1) or consecutive days (P2 and P3). Sentences had similar apparent visual length to the arithmetic equations and were presented in the same font and on the same screen background. Electrode localization We reconstructed individual three-dimensional brain images by aligning preoperative high-resolution T1-weighted magnetic resonance images (MRIs) with postoperative computed tomography (CT) scan images obtained after the electrodes implantation with an accuracy of ~±5 mm as described in our previous publications [29] , [59] , [60] , [61] . In brief, postoperative CT images were aligned to preoperative structural T1-weighted MRI whole-brain scans separately for each subject. Anatomical MRI data was reoriented to ‘AC–PC space’ by manually identifying the AC (anterior commissure), the PC (posterior commissure) and a third point in the midsagittal plane. MRI data were then resampled to 1 mm isotropic voxels using a b -spline image interpolation algorithm from SPM5 ( http://www.fil.ion.ucl.ac.uk/spm ). Postoperative CT images were then aligned to the T1 MRI anatomy scans using a mutual information algorithm from SPM5. After CT–MRI alignment, electrodes were identified in the coregistered CT image slices and their centroid coordinates recorded (subject T1 headspace). Intracranial EEG recordings Patients were implanted with flexible grid subdural platinum electrodes (AdTech Medical Instruments Corp.). The centre-to-centre interelectrode spacing was 10 mm and the diameter of each electrode’s exposed surface was 2.3 mm. Electrophysiological data were recorded simultaneously with a Tucker Davis Technologies (TDT) system and by Nihon Kohden Technology (NK) system. TDT data were synced with the display of a stimulus-presenting laptop by TTL pulses from a custom-built photodiode and NK system synced with a real-time online video camera. The TDT data were sampled at 3,052 Hz, whereas the NK data were sampled at 500 (P3) or 1,000 Hz (P1 and P2). One of the subdural electrodes served as a reference channel and an external ear lobule electrode as the ground contact for both TDT and NK systems. Preprocessing and spectral decomposition Neurologist specialized in epileptology (J.P.) examined the EEG data in all electrodes and excluded those with epileptic activity from further analysis. Notch filter from EEGLAB package ( http://sccn.ucsd.edu/eeglab ) was used to remove 60 Hz noise and its second and third harmonics. All EEG channels were re-referenced to a common average reference. EEG data were downsampled into 436 samples per second using MATLAB software. We aligned TDT and NK EEG data by calculating their maximum cross-correlation. Signals from each electrode contact were decomposed in two different ways. To make ERSP, we decomposed each channel into 42 bandwidths by filtering the signal by 42 custom-made band-pass filters. The central frequency of each band-pass filter was chosen from 1 to 232 Hz range with equal log-distance spacing. Second, each channel was also decomposed in δ (1–4 Hz), θ (4–8 Hz), α (8–12 Hz), β (15–25 Hz), low- γ (30–55 Hz) and high- γ (70–110 Hz) range by using band-pass filters from EEGLAB package. Finally, we applied Hilbert transform on decomposed signals to obtain the instantaneous amplitude of each frequency range. In this study, we call the instantaneous amplitudes of HFB range as the HFB trace. Event-related spectral perturbation The instantaneous power (square of amplitude) of each frequency was aligned and then averaged with respect to the stimulus presentation or to participant’s response time for each condition of the experiment. The trial length varied due to self-paced design of the experiment, and the number of trials in the arithmetic condition differed from the non-arithmetic condition. We matched the number of trials in the non-arithmetic condition to the arithmetic condition by choosing a subset of trials to equalize the median of trial length of both conditions. The statistical significance of power change was established by normalizing the averaged power with the mean and s.d. of the distribution of the surrogates of the entire experiment [38] . Each surrogate signal was produced by preserving the amplitude while randomizing the phase of the signal. Each time-frequency point in the surrogate ERSP matrix had a Gaussian distribution (central limit theorem) and, hence, Z -scores represented the significance of the change in power. Significance test and d ′-values The trace of power change for each lateral parietal electrode was averaged over 1 s window (from 0.5 to 1.5 s after stimulus presentation) for every trial to calculate the mean-power in six bands of δ (1–4 Hz), θ (4–8 Hz), α (8–12 Hz), β (15–25 Hz), low γ (30–55 Hz) and high- γ (70–110 Hz). We calculated the d ′- and P -values for all electrodes and for all frequency bands. Next, we normalized the mean power for each band by mean and s.d. of a generated surrogate mean-power distribution described above (the same as ERSP) by fitting the histogram of values to a Gaussian distribution with equal mean and s.d. (central limit theorem guarantees the goodness of fit). We used this mean power to test the significance of power change for each band, condition and electrode. We evaluated the null hypothesis that the mean of arithmetic trials was not different from that of non-arithmetic trials by applying non-paired Student’s t -test. We then quantified the extent to which the distribution of mean power in arithmetic trials was different from that of non-arithmetic trials by calculating the d ′-values. The d ′-value measures the distance between the means of these two distributions (centroid) in units of s.d. of non-arithmetic distribution. We sorted electrodes based on their high- γ d ′-values ( d ′ of HFB) and visualized in a mean-maximum colour scale on each patient’s three-dimensional brain as depicted in Fig. 1f . Characterization of HFB peaks To quantify the occurrence of HFB activations, we defined the so-called HFB ‘peaks’ as discrete events in the HFB traces where the HFB instantaneous amplitude increased above a chosen threshold for amplitude and was sustained beyond a chosen duration threshold. Therefore, each HFB peak was determined by two threshold parameters: amplitude and duration ( Fig. 2 ). Before searching for the optimal amplitude and duration thresholds, we smoothed the HFB traces with a standard Gaussian function (2 × σ =500 ms) to capture the local trend of HFB traces. As in the experimental task we knew which trials were arithmetic and which were non-arithmetic trials, we aimed to find the optimal values for duration and amplitude by which we could accurately identify the arithmetic trials from non-arithmetic trials. We used the ROC curve to identify the parameter that produced the highest sensitivity (hits/hits+misses) and specificity (correct rejection/correct rejection+false alarm). Hits were defined as the presence of HFB peak during arithmetic trials, misses as the absence of HFB peak during arithmetic trials, correct rejections as the absence of HFB peak in non-arithmetic trials and false alarms as the presence of HFB peak during non-arithmetic trials. The shape of the ROC curve of an electrode is determined by its d ′-value; an electrode with d ′- close to zero produces an ROC curve close to diagonal line ( Fig. 2 ). On the ROC curve, the optimal amplitude threshold is the closest point to the upper left corner (a point with the highest sensitivity and specificity). For a given electrode, we tried a range of duration values from 500 ms (the width of smoothing Gaussian function) to 1 s for a given amplitude value in a step-wise fashion ( Fig. 2a ). The ROC curve with the largest area under the curve area determined the optimal duration value. We used one of the two sessions (training) of the first experiment to find the optimal amplitude and duration thresholds. Next, we used these values to separate the arithmetic trials from non-arithmetic trials in the other session (testing) of the first experiment and in the natural condition. We use the term ‘natural condition’ even though being implanted with intracranial electrodes in a hospital may be different than the real ‘every-day’ life. Nevertheless, the daily life setting in the hospital can be considered ‘natural’, because patients were engaged in natural social interactions with other people as they would have done in any real-life setting, and our observations were made outside the artificial controlled experimental condition generated within a lab and without any obtrusive manipulations. Selectivity of HFB response We defined selectivity by the difference between HFB peak occurrence frequency during arithmetic and non-arithmetic conditions. We normalized this difference by summation of these two occurrence frequencies. We defined selectivity index as (FOA—FON)/(FOA+FON) , where FOA is the frequency occurrence of HFB peaks during arithmetic condition and FON is the frequency occurrence of HFB peaks during non-arithmetic condition. The selectivity is a value between zero (no selectivity) and one (maximum selectivity). For example, the selectivity index value of 0.25 is equivalent to 66% increase in the number of HFB peak frequency during arithmetic condition. Labelling natural events We had access to 10 (P1)- and 6 (P2 and P3)-min-long simultaneous video and intracranial EEG data from the patients when they interacted with their environment. We chose a random video segment using the following specific inclusion criteria: (1) the video should be from the same day of recording as the experimental data to avoid the plausible problem of mismatch in the signal quality between the experimental and natural files; (2) patient must interact with others and sounds must be audible (if there was no interaction between the patient and others, we could not judge the behavioural correlates of the HFB responses); and (3) lack of seizures or significant epileptic activity in the rest of the brain within 2 h before or after video file to avoid pre-ictal or post-ictal changes in the signal quality. Two independent reviewers (Stanford University undergraduate volunteers) evaluated the behavioural content of the words in conversations captured on the videos by time-stamping the start and the end of each word uttered during conversations (see Supplementary Table S1 and Supplementary Movie 1 ). Each reviewer then labelled the words that either had, or not, any numerical content. HFB peaks during numerical events in natural condition We selected videos in which the participants were awake and communicating with other people in their hospital environment. We defined the co-occurrence as the ratio of the number of HFB peaks with behavioural events in which words with numerical content were exchanged to the total number of HFB peaks during natural condition. To show that this co-occurrence ratio was not due to random alignment, we made a surrogate video by displacing the behavioural data from the end of the video to the beginning and then recalculated the co-occurrence ratio. It is noteworthy that the surrogate video data is only temporally misaligned but otherwise identical to the original video data. We made a Gaussian distribution of the co-occurrence ratio by making 500 surrogate videos. The P -value of the comparison between real and surrogate natural events is the probability of HFB peaks and numerical events being aligned by chance. We also estimated the chance level by averaging of the obtained co-occurrence values from the surrogate distribution. The sparseness of HFB peaks during natural condition The sparseness of the response during natural events was calculated by segmenting ECoG recording by non-overlapping 500 ms windows (as long as the minimum HFB peak duration). The sparseness [62] of the activity of an electrode is calculated by Sparseness={1−(∑ gi/n )^2/ ∑ ( gi^ 2/ n )}/1–1/ n }, where n is the total number of bins and gi is a bin that contains a HFB peak. The maximum sparseness is one when just one of the bins contains a HFB peak and the rest of bins are empty, and it is at minimum (zero) when all bins contain a HFB peak. How to cite this article: Dastjerdi, M. et al . Numerical processing in the human parietal cortex during experimental and natural conditions. Nat. Commun. 4:2528 doi: 10.1038/ncomms3528 (2013).